Reply to: “Steller’s sea cow uncertain history illustrates importance of ecological context when interpreting demographic histories from genomes” 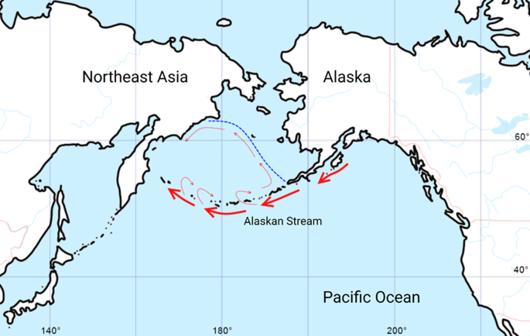Fig. 1: Simplified representation of the sea current configuration in North Pacific region. The blue dashed line schematically represents the Last Glacial Maximum coastline and the red arrows show the Alaskan Stream, which enters the Bering Sea, then forms the Aleutian North Slope (marked by red dashed arrows) current which flows into the East Kamchatka current (modified from Detlef et al.9). Further information on research design is available in the Nature Research Reporting Summary linked to this article.